Organocatalytic cycloaddition of alkynylindoles with azonaphthalenes for atroposelective construction of indole-based biaryls The axially chiral indole-aryl motifs are present in natural products and biologically active compounds as well as in chiral ligands. Atroposelective indole formation is an efficient method to construct indole-based biaryls. We report herein the result of a chiral phosphoric acid catalyzed asymmetric cycloaddition of 3-alkynylindoles with azonaphthalenes. A class of indole-based biaryls were prepared efficiently with excellent yields and enantioselectivities (up to 98% yield, 99% ee). Control experiment and DFT calculations illustrate a possible mechanism in which the reaction proceeds via a dearomatization of indole to generate an allene-iminium intermediate, followed by an intramolecular aza-Michael addition. This approach provides a convergent synthetic strategy for enantioselective construction of axially chiral heterobiaryl backbones. Axially chiral compounds are present in a plethora of natural products, biologically active compounds, and privileged chiral ligands and catalysts [1] , [2] , [3] . Consequently, developing protocols for the catalytic enantioselective construction of axially chiral scaffolds has attracted a great deal of interest among researchers in synthetic chemistry [4] , [5] . Many strategies have been developed, including desymmetrization or kinetic resolution of prochiral biaryls [6] , [7] , [8] , [9] , [10] , [11] , [12] , aryl–aryl coupling [13] , [14] , [15] , direct arylation [16] , [17] , [18] , [19] , [20] , [21] , [22] , chirality conversion [23] , [24] , [25] , [26] , [27] , [28] , [29] , [30] , [31] , [32] , [33] , cycloaddition [34] , [35] , [36] , [37] , [38] , [39] , and so on [40] , [41] , [42] , [43] , [44] , [45] , [46] , [47] , [48] . Recently, the catalytic enantioselective construction of chiral atropisomeric heterobiaryl backbones has received increasing attention from the chemistry community. However, there are still some challenges to be overcome in this field of research. Indole-based biaryls have been found in nature and have been used as ligands for asymmetric synthesis [49] , [50] , [51] . Recently, a few outstanding cases of the enantioselective synthesis of indole–aryl skeletons have been reported [22] , [29] , [33] , [52] , [53] , [54] , [55] , [56] , [57] , [58] , [59] , [60] , [61] , [62] , [63] , [64] , [65] , [66] . Generally, there are two strategies to construct indole-based biaryls enantioselectively. One is asymmetric coupling reaction of indole derivatives with other aryls [22] , [56] , [57] , [58] , [59] , [60] , [61] , [62] , the other is in situ construction of indole skeletons atroposelectively [63] , [64] , [65] , [66] . Interestingly, o -alkynylanilines were usually employed for the synthesis of indoles possessing chiral axis by the latter strategy. For instance, Kitagawa and coworkers reported an elegant Pd(II)-catalyzed enantioselective hydroamination reaction to construct indoles bearing an N-aryl chiral axis [53] , [55] . Li and coworkers merged C−H activation with nucleophilic cyclization to realize oxidative coupling of indoles and o -alkynylanilines for the synthesis of biindolyls [63] . Zhu and coworkers developed a palladium-catalyzed asymmetric Cacchi reaction for the construction of indoles bearing a chiral axis [66] . Yan and coworkers established an organocatalytic enantioselective construction of chiral indole-aryl skeletons through an asymmetric annulation [64] . Notably, the intramolecular annulation strategy, a linear synthesis has been adopted to form a single C–N bond to generate the indole skeleton in all these protocols (Fig. 1a ). While the intermolecular strategy, a convergent synthesis strategy for the atroposelective construction of indole–aryls remains limited. Therefore, to realize a divergent synthesis of such indole-based biaryls, designing of more efficient strategies is of great significance. Fig. 1: Asymmetric construction of indole-based biaryls via cycloaddition strategies. a Construction of indole derivatives via intramolecular cyclization. b CPA-catalyzed atroposelective intermolecular [3 + 2] cycloaddition. Full size image In fact, transition metal catalyzed cyclization reaction of azobenzene derivatives with alkynes to construct indole derivatives without chiral axis has been reported [67] , [68] , [69] . Although organo-catalyzed cycloaddition of alkenes with azonaphthalenes has been well documented [22] , [29] , [33] , [70] , the organo-catalyzed asymmetric cycloaddition reaction of azo benzene derivatives with alkynes is still lacking. The reason may be ascribed to a relative lower reactivity of alkyne than that of alkene in the cycloaddition reaction with azonaphthalenes. We envisioned that installation of electron-donating groups to alkyne moiety would enhance such reactivity, and further activated by organocatalyst would realize the desired cycloaddition to give the corresponding indole–aryl atropisomers. In order to achieve this goal, we needed to overcome the following issues: (1) realization of efficient annulation of alkynes with azonaphthalenes; (2) the installation of a suitable group onto the 1-ethynylnaphthene to avoid free rotation around the C–C axis; (3) the choice of a competent chiral catalyst to activate reaction partners and to control the stereoselectivity. Herein, we report a formal [3 + 2] cycloaddition strategy for atroposelective construction of indole-based biaryls via chiral phosphoric acid (CPA)-catalyzed cycloaddition reaction of 3-alkynylindoles with azonaphthalenes (Fig. 1b ). We commenced the reaction of 1-ethynylnaphthol with azonaphthalene to examine the possibility of our strategy. 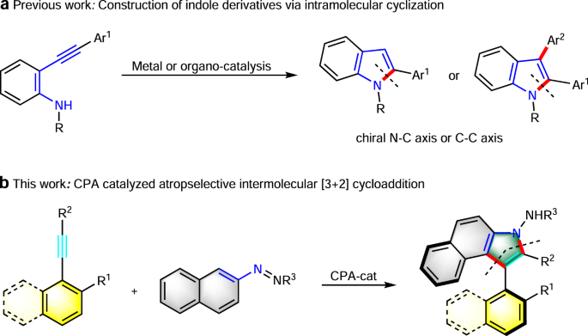Fig. 1: Asymmetric construction of indole-based biaryls via cycloaddition strategies. aConstruction of indole derivatives via intramolecular cyclization.bCPA-catalyzed atroposelective intermolecular [3 + 2] cycloaddition. Unfortunately, no reaction occurred when a series of reaction conditions were attempted (for details, see Supplementary Table 1 ). The reason may be due to that the electron density of the alkyne was still insufficient to perform the nucleophilic addition to azonaphthalenes. Then we changed the naphthols with more electron-rich indoles, 3-alkynylindol derivatives as the substrate. To our delight, the desired cycloaddition products could be obtained smoothly. As shown in Table 1 , chiral phosphoric acid 16a (10 mol%) catalyzed the reaction of 3-alkynylindole 1a with azonaphthalene 8a in toluene at −50 o C for 72 h, the desired cycloaddition product 9a was obtained in moderate yield and enantioselectivity (entry 1). An increase in enantioselectivity was realized when catalyst 16b was used (entry 2). The CPA 16c , bearing a 9-phenanthryl group at the 6,6′-position of SPINOL, provided the desired product 9a with good yield and enantioselectivity (87%, 86% ee, entry 3). Having realized the efficiency of the annulation, we turned our effort to improve the enantioselectivity. First, the installation of suitable protection groups onto the naphthol of 3-alkynylindole derivatives was performed to avoid free rotation around the C–C axis during the reaction. As expected, the enantioselectivity declined to around 40% when methoxymethyl was substituted with a less bulky methyl group (entry 4). On the other hand, the more bulky group benzyl or tert -Bu has an enhancing effect on the enantioselectivity, albeit with the reaction efficiency was dramatically decreased, probably due to the steric reason (entries 5,6 vs entry 4). These results demonstrated that the R group plays an important role in the stereocontrol in this reaction. The use of substrate 5a containing a cyclohexyl group could afford the corresponding product in 65% yield with 87% ee (entry 7). Interestingly, iso -Pr returned the desired product in 95% yield with 90% ee (entry 8). Moreover, 7a bearing a 3-pentyl group was found to be the optimal substrate, affording the desired product 15a in good yield and excellent enantioselectivity (75%, 94% ee, entry 9). Further optimization of the reaction by a variety of solvents (CH 2 Cl 2 , CH 3 CN, CCl 4 , and CHCl 3 ) was subsequently investigated (entries 10–13), and CHCl 3 gave the best result (97% ee, entry 13). In addition, a further decrease of the reaction temperature could not improve the enantioselectivity of the reaction (entry 14). Meanwhile, increasing the temperature to −25 o C or 0 o C has a negative effect on the reaction transformation (entries 15–16). Fortunately, when the catalyst loading was reduced to 5 mol% or 2 mol%, the enantioselectivity almost remained unchanged and excellent yields were still obtained (entries 17–18). Further reducing the amount of the catalyst to 1 mol% resulted in a measurable decrease in the yield (entry 19). The thermal racemization of these atropisomers was conducted to investigate the configurational stability (for details, see Supplementary Information). Compound 15a displays an excellent stability with a barrier to enantiomerization of 173 kJ mol −1 , and the half-life time of racemization was determined to be 3.3 × 10 9 years at 25 o C. Table 1 Optimization of the reaction conditions a . Full size table With the optimal reaction conditions in hand, we examined the substrate scope of the protocol (Fig. 2 ). First, the substitution effect at the indole was examined. Substituents of the phenyl ring of the indole core with halogens at the 5-position, such as F, Cl, and Br, afforded the corresponding axially chiral products with excellent yields and enantioselectivities ( 15b–d , 90–96%, 97–98% ee). The methyl or methoxy-group substituent at the 5-position of the indole could be well tolerated to give the expected products 15e and 15f , respectively, with excellent results (up to 98% yield, 98% ee). In addition, product 15g with a 5-Ph substituent indole was obtained in 75% yield and 96% ee. The halogen (F, Cl, and Br)-containing substrates at the 6-position of the indole were tolerated under the standard conditions, all proceeding in excellent yields and enantioselectivities ( 15h–j , 97–98%, 95–97% ee). Substrates with the substituents CH 3 and Ph at the 6-position of the indole all resulted in the corresponding desired products with good yields and excellent enantioselectivities ( 15k , 15l , 97% ee). A 7-chloro-substituted indole substrate 7m returned an 87% yield with 98% ee. Interestingly, when chloro substituent was installed at the 4-position of the indole, the corresponding product 15n bearing two stereogenic axes was obtained in good yield with excellent enantioselectivity and moderate diastereoselectivity. Substrate 7o was also used to construct the compound containing two stereogenic axes, unfortunately, poor stereoselectivity was observed. Fig. 2: Substrate scope. a Reactions were carried out with 7 (0.24 mmol), 8 (0.20 mmol), and 16c (0.004 mmol) in CHCl 3 (2.0 mL) at −50 °C under N 2 . The yields shown are for isolated products and the ee values were determined by HPLC analysis. b The reaction temperature is 40 °C. Full size image Next, we examined the substrate scope with regard to the naphthyl ring moiety and other azonaphthalenes. 3-Pentan-3-yloxy at the 3-position of the naphthyl ring resulted in the desired product 15p in 80% yield with 93% ee. Different substituents at the 6-position of the naphthyl ring, such as CH 3 , Br, and Ph all could afford the desired products in good yields and excellent enantioselectivities ( 15q–s , 73–98% yields, 97–98% ee). Moreover, both electron-rich and electron-deficient substituents at the 7-position of the naphthyl ring returned the desired axially chiral compounds in up to 97% yield with up to 99% ee ( 15t–v ). On the other hand, the substrates with different substituents at the 6 or 7-position of the azonaphthalene were well tolerated and delivered the corresponding products 15w–z in high yields (63–95%) and excellent enantioselectivities (92–99% ee). Among them, the product 15y was obtained in 63% yield and 93% ee at 40 °C. Finally, azonaphthalene with different N-protecting groups could be employed, delivering the corresponding axially chiral products in moderate-to-good yields (52–83%) and excellent enantioselectivities ( 15aa–ae , 94–97% ee). Besides naphthyl-substituted alkynylindole, phenyl-substituted alkynylindole 7af was also treated under the optimal reaction conditions, satisfyingly, the desired axially chiral product 15af was obtained in 79% yield and 80% ee. The relatively lower enantioselectivity may be due to its lower configurational stability. Indeed, compound 15af displays a lower stability with a barrier to enantiomerization of 100 kJ mol −1 , and the half-life time of racemization was determined to be 4.8 hours at 25 o C (for details, see Supplementary Information). The absolute configuration of the product was assigned on the basis of the X-ray crystallographic structure of 15x . Interestingly, compound 15ag bearing two chiral axes can be generated with 94% ee by this strategy starting from 7ag , albeit a lower yield (Fig. 3 ). To test the practicality of this method, a gram-scale reaction of 7a with 8a was carried out under the standard reaction conditions. As expected, compound 15a was obtained successfully with excellent yield and enantioselectivity (Fig. 4a ). In addition, reduction of 15a with LiAlH 4 provided the secondary amine product 17 in good yield and no changes occurred in the stereoselectivity during this reaction. The 3-pentyl group could also be removed smoothly by using BBr 3 in CH 2 Cl 2 for 4 h, giving phenol product 18 in quantitative yield without any loss of enantiopurity, which is a useful building block for further transformation. Trifluoromethylation of 18 afforded product 19 in excellent yield and enantioselectivity (95% yield, 97% ee), which is a potential partner in metal-catalyzed coupling reactions (Fig. 4b ). The protecting group on the azonitrogen center could be removed, affording compound 20 in good yield. The axially chiral benzoindolenaphthyl-derived thiourea compound 21 bearing 3,5-bis(trifluoromethyl)phenyl group was prepared smoothly in 90% yield according to the classical approach for the preparation of cinchona-derived thiourea catalyst (Fig. 4c ). Fig. 3: Construction of diaxial compound 15ag. The reaction was carried out with 7ag (0.05 mmol), 8a (0.125 mmol), and 16c (0.002 mmol) in CHCl 3 (0.5 mL) at −50 °C under N 2 . Full size image Fig. 4: Gram-scale synthesis and transformations. a Gram-scale synthesis of axially chiral compound 15a . b Transformation of compound 15a . c Synthesis of axially chiral organocatalyst. Full size image On the basis of the above transformation, we attempted to transform compound 15a into potential useful phosphine ligands to showcase the practical value of the products. As shown in Fig. 5 , treatment of 20 with [Ir[dF(CF 3 )ppy] 2 (dtbbpy)PF 6 ] catalyst under 5w blue LED lamp, in CH 3 OH/CH 3 CN provided 22 . Compound 24 was prepared from 22 , and the enantioselectivity was retained even after three steps (98% ee). Finally, compound 24 was transformed into the benzoindolenaphthyl phosphine ligand 25 by reduction with HSiCl 3 reagent. A preliminary application of 25 (98% ee) as ligand in the asymmetric allylation reaction of ( E )-1,3-diphenylallyl acetate with dimethyl malonate revealed that 25 is efficient at promoting the reaction (99% yield), although the enantioselectivity of product 28 needs to be improved (39% ee). Fig. 5: Synthesis and application of chiral phosphine ligand. a Synthesis of chiral phosphine ligand 25 . 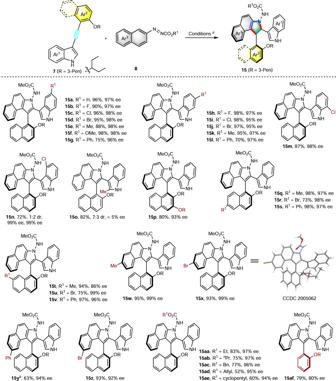Fig. 2: Substrate scope. aReactions were carried out with7(0.24 mmol),8(0.20 mmol), and16c(0.004 mmol) in CHCl3(2.0 mL) at −50 °C under N2. The yields shown are for isolated products and the ee values were determined by HPLC analysis.bThe reaction temperature is 40 °C. b Asymmetric allylation using 25 as the ligand. Full size image To get mechanistic insights into this reaction, a control experiment was carried out under the optimal conditions. 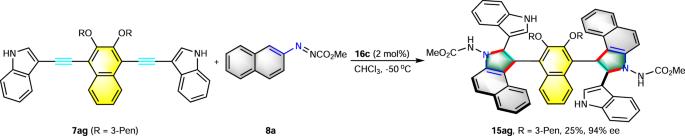Fig. 3: Construction of diaxial compound 15ag. The reaction was carried out with7ag(0.05 mmol),8a(0.125 mmol), and16c(0.002 mmol) in CHCl3(0.5 mL) at −50 °C under N2. 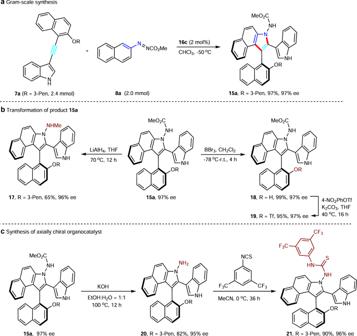Fig. 4: Gram-scale synthesis and transformations. aGram-scale synthesis of axially chiral compound15a.bTransformation of compound15a.cSynthesis of axially chiral organocatalyst. The desired product could not be obtained when the N–H group of 7a was protected with methyl, which demonstrated that the N–H group plays an important role in the process. To better understand the mechanism and origins of stereo- and regioselectivity, density-functional theory (DFT) calculations were conducted using Gaussian 09 program. All the intermediates and transition states were optimized by employing the xc-functional ωB97X-D with dispersion correction (ωB97X-D) and the 6-31G(d) basis set. Normal vibrational mode analysis at the same level of theory confirmed that the optimized structures are minima (zero imaginary frequency) or saddle points (one imaginary frequency). Based on optimized geometries, single-point energies and solvent effects in chloroform were computed with the range-separated functional ωB97X-D and the 6-311G (d,p) basis set using the SMD model. To save computational time, the phenanthryl moieties in the catalyst were replaced with methyls and 3-pentyl in the substrate with methyl. The free-energy profiles (in kcal/mol) of the most favorable pathway for the phosphoric acid-catalyzed cycloaddition of alkynylindoles with azonaphthalenes are shown in Supplementary Fig. 2 . First, the chiral phosphoric acid acts as a bifunctional catalyst to simultaneously activate 3-alkynylindoles and azosubstrates through a dual hydrogen-bonding activation mode to generate a complex. Subsequent dearomatization of 3-substituted indole generates the transient allene-iminium intermediate [62] , [71] , [72] , [73] , [74] , which further undergoes an intramolecular aza-Michael addition to afford the axially chiral intermediate. 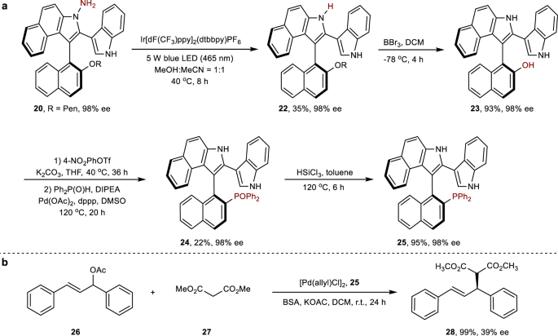Fig. 5: Synthesis and application of chiral phosphine ligand. aSynthesis of chiral phosphine ligand25.bAsymmetric allylation using25as the ligand. Finally, deprotonation and aromatization yields the desired product. 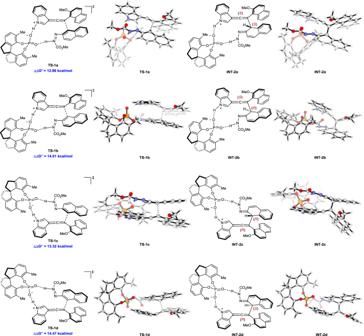Fig. 6: DFT calculations. DFT-optimized chiral phosphoric acid-catalyzed transition statesTS-1a–d, and their corresponding allene–iminium intermediatesINT-2a–d. Figure 6 shows the optimized structures and relative free energies of the four competing stereoselectivity-determining allene–iminium transition states TS-1a , TS-1b , TS-1c , and TS-1d , and the structures of their corresponding allene–iminium intermediates. Indeed, the calculated re -face attack TS - 1a is found to be 3.7 kcal/mol lower in the relative free energy than the si -face attack in TS - 1b . The potential energy of the allene–iminium intermediate INT-2a was also found to be lower than that of the intermediate INT-2b by 0.89 kcal/mol (for details, see Supplementary Information). Transition states TS - 1a and TS - 1c would generate S - and R -configuration product, respectively. The relative activation-free energy (ΔΔG) for TS - 1a is 12.98 kcal/mol more favorable than TS - 1c , which corroborated the observed enantioselectivity that the ( S )-selective product was obtained. In addition, the TS-1a that ultimately leads to the major conformation product is 6.22 kcal/mol more stable than TS-1d , which is in good agreement with the experimental result. Fig. 6: DFT calculations. DFT-optimized chiral phosphoric acid-catalyzed transition states TS-1a–d , and their corresponding allene–iminium intermediates INT-2a–d . Full size image In this work, we show the CPA-catalyzed intermolecular [3 + 2] formal cycloaddition of 3-alkynylindoles with azonaphthalene for the enantioselective construction of indole-based atropisomers. A type of axially chiral arylindole derivatives were afforded in high yields and excellent stereoselectivities (up to 98% yield, 99% ee). In addition, this transformation allows lowering of the catalyst loading to 2 mol% without considerable loss of reactivity and enantioselectivity. This reaction not only provides a useful method for constructing enantioenriched indole-based biaryl atropisomer scaffolds, but also advances the chemistry of catalytic asymmetric reactions of alkynylindoles. General procedure for the enantioselective synthesis of 15 To a stirred solution of 7 (0.24 mmol), 8 (0.20 mmol) and CPA 16c (0.004 mmol) in CHCl 3 (2.0 mL) at −50 °C in one portion, the mixture was stirred until TLC revealed the absence of the starting material. The solvent was removed under reduced pressure, the residue was purified by flash-column chromatography (petroleum ether/EtOAc) to yield the corresponding product 15 . Synthesis of 18 To a mixture of 15a (113 mg, 0.2 mmol, 1.0 eq) in CH 2 Cl 2 (2 mL) at −78 °C was added BBr 3 (0.2 mL, 1.0 mol/L CH 2 Cl 2 , 1.0 eq) dropwise, and the mixture was stirred for 4 hours at room temperature. TLC showed complete consumption of the starting material. The reaction was quenched with 10% NaHCO 3 solution and extracted with CH 2 Cl 2 (3 × 5 mL). The combined organics were washed with brine and dried over Na 2 SO 4 . The solvent was removed under reduced pressure, the residue was purified by column chromatography on silica gel (20% EtOAc in hexane) to yield 18 as a white solid (98.4 mg, 99% yield). Synthesis of 19 The reaction was performed using 18 (98.4 mg, 0.2 mmol, 1.0 eq), 4-nitrophenyl trifluoromethanesulfonate (65 mg, 0.24 mmol, 1.2 eq), and K 2 CO 3 (41.5 mg. 0.3 mmol, 1.5 eq) in THF (2.0 mL) at 40 o C. After finishing, the reaction was quenched with H 2 O (5 mL). The solution was extracted with CH 2 Cl 2 (3 × 5 mL), washed with brine (5.0 mL), and dried over anhydrous Na 2 SO 4 . The solvent was evaporated under reduced pressure. The crude product was purified by flash-column chromatography (10% EtOAc in hexane) giving 19 as a white solid (119.5 mg, 95% yield).